Cobalt-catalyzed atroposelective C−H activation/annulation to access N−N axially chiral frameworks The N−N atropisomer, as an important and intriguing chiral system, was widely present in natural products, pharmaceutical lead compounds, and advanced material skeletons. The anisotropic structural characteristics caused by its special axial rotation have always been one of the challenges that chemists strive to overcome. Herein, we report an efficient method for the enantioselective synthesis of N−N axially chiral frameworks via a cobalt-catalyzed atroposelective C-H activation/annulation process. The reaction proceeds under mild conditions by using Co(OAc) 2 ·4H 2 O as the catalyst with a chiral salicyl-oxazoline (Salox) ligand and O 2 as an oxidant, affording a variety of N−N axially chiral products with high yields and enantioselectivities. This protocol provides an efficient approach for the facile construction of N−N atropisomers and further expands the range of of N−N axially chiral derivatives. Additionally, under the conditions of electrocatalysis, the desired N−N axially chiral products were also successfully achieved with good to excellent efficiencies and enantioselectivities. Atropisomerism, as one kind of intriguing axial chirality, has greatly aroused explosive attention due to their fascinating architectures and excellent multidisciplinary applications (pharmaceutical exploitation, functional materials development), arising from the restricted rotation around a single bond [1] , [2] , [3] , [4] , [5] . Since the pioneering work by Kenner on the expound of axial chirality from the perspective of fabrication and development significance via organic synthetic tactics in early 19th century [6] , innumerable atropisomerism-based skeletons have been continually discovered due to the continuous progress in preparation, separation, purification methods and instruments. In this context, C–C and C–N atropisomers, including axially chiral biaryls, aryl amines, and aryl amides, are emerging at an amazing speed, and a variety of innovative achievements have been sparkled over the past two decades [7] , [8] , [9] , [10] , [11] , [12] , [13] , [14] , [15] , [16] , [17] , [18] , [19] . The atropisomerism of N–N bond, however, eluded such serious attention for a long time, which might be attributed to the incorrect notion that N–N axis is unstable due to the deplanarization effect. Indeed, the electronic barrier stemming from the repulsive interaction between the lone pairs on the two nitrogen atoms can strongly favor the formation of such atropisomers. These intriguing atropisomerism configurations have moved onto the research stage again due to the new structural understanding, making them a superior platform for serving N–N axial natural products, bioactive molecules, functional materials, and ligands production (Fig. 1a ) [20] , [21] , [22] , [23] , [24] , [25] . By contrast, the atropisomerism bearing a N–N bond remains largely underdeveloped, possibly due to the shorter length and weaker nature of the N–N bond [26] . Besides, the low rotational barrier caused by the two N -containing planes deplanarization, renders the N–N axis construction more challenging. Typically, the N–N axially chiral skeletons could be built up through four types of transformations (Fig. 1b ). The atroposelective N–H functionalization, such as allylation, alkylation, and acylation, represents an effective mean by modifying the central N–N axis [27] , [28] , [29] , [30] . Alternatively, catalytic asymmetric desymmetrization of pro-chiral substrates [31] , [32] , and asymmetric assembly via de novo construction of pyrroles and indoles [33] , [34] , [35] , [36] , [37] also provide satisfactory choices for creating N–N atropisomers. Typically, Shi group have recently achieved organocatalytic enantioselective construction of N–N axially chiral indoles and pyrroles [36] , [37] . More recently, Liu and You groups successfully reported the construction of N–N atropisomers via the Pd or Ir-catalyzed C–H functionalization of indole/pyrrole ring through dynamic kinetic resolution of racemic N–N biaryls [38] , [39] , further advancing the development of this field. Despite the elegant efforts made, research in this area is still in its infancy and remains underdeveloped. As a result, the development of more efficient and facile approaches for building novel and diverse N–N atroposelective frameworks is highly appealing yet challenging. Fig. 1: Background and project synopsis. a Representative molecules bearing an N–N axis. b Synthetic strategies for N–N atropisomers. c This work: Co/Salox-catalyzed atroposelective C–H activation/annulation. Full size image For this purpose, asymmetric C–H functionalization, as a timely emerged and well-established tactic, was built up to form diverse charming structures containing highly functionalized skeletons, such as natural products, pharmaceutical lead compounds, important architectures which typically takes advantage of batch production with satisfactory chemical selectivity (stereoelectronic selectivity and regioselectivity) via transition metal catalyzed process [40] , [41] , [42] , [43] , [44] , [45] . In this content, the first-row 3d-metal cobalt-catalyzed C–H functionalization has gained increasing popularity owing to its earth-abundance, low toxicity, and distinctive reactivities [46] , [47] , [48] , [49] , [50] , [51] , [52] , [53] , which has been largely developed for the synthesis of various skeletons by Ackermann [54] , [55] , [56] , Yoshino and Matsunaga [57] , [58] , [59] , [60] , Cramer [61] , [62] , [63] , Shi [64] , [65] , [66] , [67] , [68] , [69] , and our groups [70] , [71] , [72] , [73] . Very recently, our group [70] , and Shi’s group [65] independently developed an efficient chiral Co/Salox (salicyl-oxazoline) system, and demonstrated its excellent reactivity for assembling C–N and C–C axially chiral compounds. This strategy features significant advantages, making easily available cobalt salt catalyzed C–H functionalization for constructing axial chiral compounds being a promising research area. On the other hand, the nitrogen atoms in the N–N atropisomers may be derived from different substructures, giving rise to the possibility of forming diverse N–N axially chiral compounds. However, to the best of our knowledge, the construction of N–N axially chiral atropisomers via earth abundant transition-metal catalyzed C–H activation remains unprecedented. Inspired by the elegant and well-established cobalt-catalyzed C–H activation/functionalization developments, and with our continuing interest in cobalt catalysis, we hope to achieve further development in this field through the strategy of direct asymmetric C–H activation. Delightedly, we here reported a highly efficient example of cobalt-catalyzed atroposelective construction of N–N axially chiral frameworks, combining the advantages of excellent efficiency and enatioselectivities (up to 98% yield and 99% e.e.) based on cobalt/Salox catalysis, which undoubtfully broaden the synthetic strategies for the direct and effective construction of N–N atropisomers and further enrich the types/scopes of N–N axially chiral derivatives. This approach has proved to be a highly suitable way for efficient preparation of N–N atropisomers according to their readily available raw materials, and accessible operation characteristics (Fig. 1c ). Notable features of this protocol include: (1) the cheap cobalt(II) salt enabled N–N chiral axis construction, (2) the use of environmentally friendly O 2 as the oxidant, (3) high yields and excellent enantioselectivities with good functional group tolerance, (4) successful application under electrochemical conditions, (5) the unique atropostability for the N–N axially chiral products. 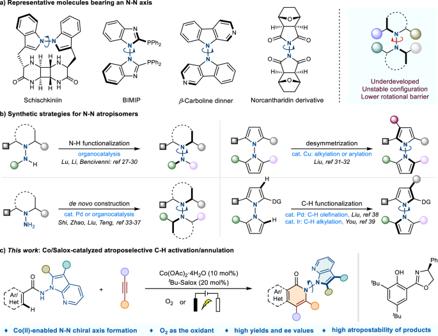Fig. 1: Background and project synopsis. aRepresentative molecules bearing an N–N axis.bSynthetic strategies for N–N atropisomers.cThis work: Co/Salox-catalyzed atroposelective C–H activation/annulation. Optimizing reaction conditions To validate the feasibility of the hypothesis, our investigation was initiated by using the N -(7-azaindole)benzamide 1a and phenylacetylene 2a as the model substrates, with 10 mol% of Co(OAc) 2 ·4H 2 O as the catalyst and O 2 as the oxidant (Table 1 ). Diverse chiral Salox ligands L1 – L7 were evaluated. It was pleased to find that the desired N–N axially chiral isoquinolinone product 3aa was obtained with 48% yield and excellent 99% ee, with L6 bearing bulky tert -butyl groups at the ortho - and para -position of phenol as the chiral ligand. And this promoting effect of the bulky t Bu-Salox ligand has also been reported in the previous Co/Salox catalysis developed by Shi [69] , Ackermann [56] and our group [73] . 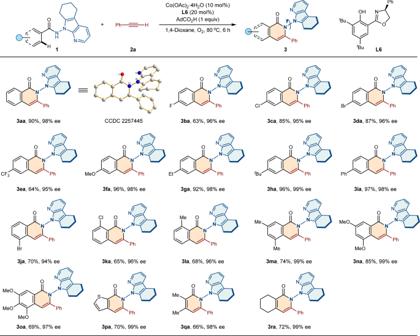Fig. 2: Scope of benzamides. Reaction conditions:1(0.2 mmol),2a(0.24 mmol), Co(OAc)2·4H2O (0.02 mmol),L6(0.04 mmol), AdCO2H (0.2 mmol) in 1,4-dioxane (2 mL) at 80 °C under O2for 6 h, isolated yields. ee, enantiomeric excess. Various cobalt catalysts, such as Co(OAc) 2 , and Co(OBz) 2 , CoCl 2 ·6H 2 O, were fully investigated, in which no better results have got (entries 1–4, and Supplementary Table 2 ). 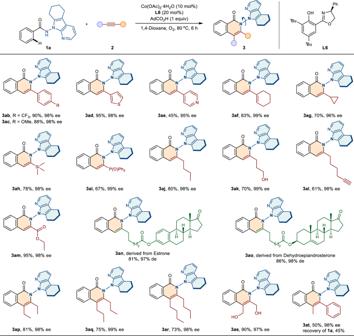Fig. 3: Scope of alkynes. Reaction conditions:1a(0.2 mmol),2(0.24 mmol), Co(OAc)2·4H2O (0.02 mmol),L6(0.04 mmol), AdCO2H (0.2 mmol) in 1,4-dioxane (2 mL) at 80 °C under O2for 6 h, isolated yields. de, diastereomeric excess. The effects of the solvent were then screened, and 1,4-dioxane displayed the best activity (entries 5–8, and Supplementary Table 3 ). 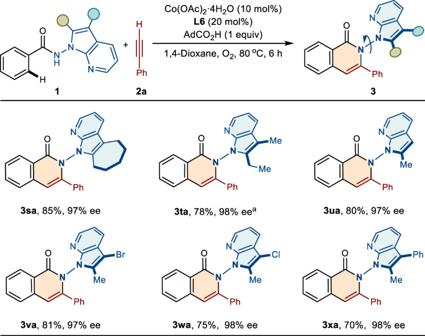Fig. 4: Scope of Benzamides with Substituents on the 7-Azaindole Ring. Reaction conditions:1(0.2 mmol),2a(0.24 mmol), Co(OAc)2·4H2O (0.02 mmol),L6(0.04 mmol), AdCO2H (0.2 mmol) in 1,4-dioxane (2 mL) at 80 °C under O2for 6 h, isolated yields.a20 mol% Co(OAc)2·4H2O, 10 h. ee enantiomeric excess. Further optimization was conducted by the use of additives, such as NaOPiv·H 2 O, AcOH, and AdCO 2 H (entries 9–11, and Supplementary Table 4 ), and AdCO 2 H proved to be the best choice. Further optimization of the reactive temperature, time, and catalyst/ligand loadings, revealed that the reaction was able to produce the atroposelective isoquinolinone 3aa with 94% yield and 98% ee at 80 o C for 6 h (entries 12–13, and Supplementary Tables 5 – 8 ). The absolute configuration of N–N axially chiral 3aa was determined to be R a by X-ray diffraction analysis (CCDC 2257445). In addition, a competitive experiment by using 1a and 1a’ bearing a 7-methyl-8-aminoquinoline directing group with a 1:1 ratio as substrate was conducted under optimized conditions, and the product 3aa and 3aa’ were obtained with a total yield of 99% with a 1:1 ratio (See Supplementary Table 10 ). Table 1 Optimization studies a Full size table Substrate scope With the optimal conditions in hand, we then explored the substrate generality of this transformation (Fig. 2 ). A variety of benzamides with diverse functionalities at para -position were systematically investigated. To our delight, both electron-withdrawing (−F, −Cl, −Br and −CF 3 ) and electron-donating (−OMe, −Et, − t Bu, and −Ph) groups were well tolerated to afford the N–N axially chiral isoquinolinones 3ba − 3ia in good yields (63–97%) and excellent enantioselectivities (95 − 99% ee). For the meta -substituted substrate 1j , the annulation took place at the sterically more hindered position to provide 3ja in 70% yield and 94% ee. Ortho -substituted benzamides 1k and 1l also reacted smoothly, delivering 3ka and 3la with good yields and high enantiopurities of 96% ee. When multi-functionalized substrates with methyl or methoxy substituents located at the aromatic ring, the desired N–N axially chiral isoquinolinones 3ma − 3oa could also be obtained with good to excellent efficiencies and enantioselectivities. Notably, the heterocyclic substrate 1p containing a thienyl moiety also reacted smoothly to give the product 3pa with 70% yield and 99% ee. In addition, the challenging vinylamides 1q and 1r were well compatible with this atroposelective transformation, delivering products 3qa and 3ra with high level of enantiocontrol (98–99% ee). Fig. 2: Scope of benzamides. Reaction conditions: 1 (0.2 mmol), 2a (0.24 mmol), Co(OAc) 2 ·4H 2 O (0.02 mmol), L6 (0.04 mmol), AdCO 2 H (0.2 mmol) in 1,4-dioxane (2 mL) at 80 °C under O 2 for 6 h, isolated yields. ee, enantiomeric excess. Full size image Alkyne substrates were further expanded to verify the generality of the protocol. As shown in Fig. 3 , both electron-donating (−OMe) and electron-withdrawing (−CF 3 ) groups at the para -position of phenylacetylene were well tolerated, and the corresponding products 3ab and 3ac were obtained in 90 yield, 98% ee and 88% yield, 98% ee, respectively. The heterocycle-substituted alkynes (including 3-ethynylthiophene and 4-ethynylpyridine), conjugated enyne, and cyclopropyl acetylene were also found to be compatible with this reaction, furnishing the desired products 3ad − 3ag with excellent enetioselectivities (95–99% ee). Notably, the presences of Si and P substituents in the resulting N–N axially chiral products ( 3ah − 3ai ) were particularly important for further derivation owing to their inherent reactivity. In addition, the alkyl or ester-substituted terminal alkynes, even with functional groups, proved to be suitable coupling partners to give products 3aj − 3am with good yields (61–95%) and high enantiopurities (98 − 99%). To further demonstrate the practicality of the protocol, the natural product-linked alkynes 2n and 2o were synthesized and utilized for the related atroposelective annulation, and the target products were successfully obtained in 81–86% yields and high diastereomeric excess (97–98% de). Moreover, the aliphatic internal alkynes 2p − 2s also reacted smoothly to deliver N–N axially chiral isoquinolinones 3ap − 3as with 97–99% ee values. For the unsymmetrical internal alkyne 2t , the reaction proceeded with exclusive regioselectivity to give 3at in moderate yield and high enantioselectivity, and the starting material of 1a was recovered with a 45% yield. But the diphenylacetylene was incompatible in this system, possibly due to the steric hindrance. Fig. 3: Scope of alkynes. Reaction conditions: 1a (0.2 mmol), 2 (0.24 mmol), Co(OAc) 2 ·4H 2 O (0.02 mmol), L6 (0.04 mmol), AdCO 2 H (0.2 mmol) in 1,4-dioxane (2 mL) at 80 °C under O 2 for 6 h, isolated yields. de, diastereomeric excess. Full size image Subsequently, the scope of the benzamides bearing different substituents on the 7-azaindole ring were investigated. As shown in Fig. 4 , for azaindole backbone, which was functionalized by cyclohexane moiety, was well compatible, generating 3sa in good yield (85%) and high enantiopurity (97% ee). The protocol also tolerated 2-ethyl and 2-methyl substituted azaindoles, furnishing the desired products 3ta and 3ua with high enantiocontrol (98% ee and 97% ee, respectively). In addition, benzamides bearing functionalities located on the C2 and C3 position of the azaindole ring, reacted smoothly to deliver N–N axially chiral products 3va - 3xa , with good reactivities (70–81% yields) and excellent enantioselectivities (97–98 % ee). Fig. 4: Scope of Benzamides with Substituents on the 7-Azaindole Ring. Reaction conditions: 1 (0.2 mmol), 2a (0.24 mmol), Co(OAc) 2 ·4H 2 O (0.02 mmol), L6 (0.04 mmol), AdCO 2 H (0.2 mmol) in 1,4-dioxane (2 mL) at 80 °C under O 2 for 6 h, isolated yields. a 20 mol% Co(OAc) 2 ·4H 2 O, 10 h. ee enantiomeric excess. Full size image To gain more efficiencies into the reactive practicality, related electrochemical experiments were conducted (Fig. 5 ). The general substrates were also compatible to afford the corresponding N–N axially chiral isoquinolinones 3aa and 3ia without any reduction of enantioselectivities. For silicon and dialkyl substituents based on alkynes, the current protocol also proved to be a powerful tactic for diverse N–N axially chiral frameworks ( 3ah and 3aq ). Fig. 5: Reaction scope for the electro-oxidative annulation. Reaction conditions: graphite felt anode, Pt-plate cathode, constant current = 2 mA, 1 (0.2 mmol), 2 (0.24 mmol), Co(OAc) 2 ·4H 2 O (0.02 mmol), L7 (0.04 mmol), TFE (5 mL), NaOPiv·H 2 O (0.4 mmol), 60 o C, 6 h, air, isolated yields. ee, enantiomeric excess; TFE, 2,2,2-trifluoroethanol. Full size image Study on product stability and synthetic applications To further explore the conformational stability of N–N axially chiral isoquinolinones, the racemization experiments were investigated (Fig. 6 ). Initially, the newly formed 3aa was heated up to 160 °C in dodecane, and the ee value can be maintained without decreasing. The ee value of 3aa decreased by 0.53% after 10 h at 180 °C. And the rotational energy barrier of 3aa was calculated to be 41.6 kcal/mol, and its half-life ( t 1/2 ) was up to 5.5 × 10 9 years at 25 °C. As the experimental results shown, energy barrier and the t 1/2 of 3aq and 3ua were also exhibited, indicating that the N–N axially chiral isoquinolinones endowed a high degree of atropostabilities. It is worth noting that the compounds 3aa, 3aq , and 3ua underwent slight decomposition after being heated for 6 or 10 h. And the recovery rates for 3aa, 3aq , and 3ua were 70%, 60%, and 90%, respectively. To verify the accuracy of the testing rotational energy barriers, we further studied the enantiomerization processes of 3aa and 3ua by DFT calculations. As shown in Fig. 6 and Supplementary Fig. 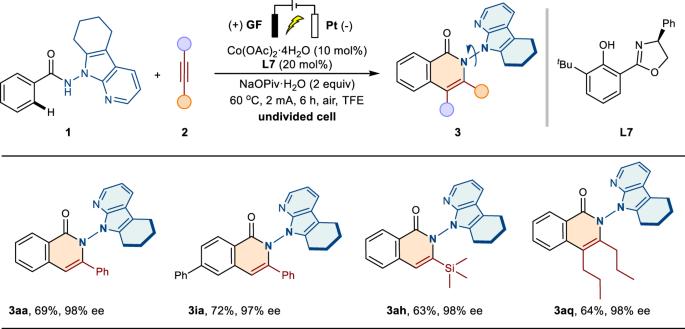Fig. 5: Reaction scope for the electro-oxidative annulation. Reaction conditions: graphite felt anode, Pt-plate cathode, constant current = 2 mA,1(0.2 mmol),2(0.24 mmol), Co(OAc)2·4H2O (0.02 mmol),L7(0.04 mmol), TFE (5 mL), NaOPiv·H2O (0.4 mmol), 60oC, 6 h, air, isolated yields. ee, enantiomeric excess; TFE, 2,2,2-trifluoroethanol. 6 , the energy barriers of the dihedral rotation via transition states TS 3 aa and TS 3 ua are 40.3 kcal/mol and 41.2 kcal/mol respectively, which showed good agreement with the experimental results. Fig. 6: Study on product stability. The rotation barrier and the t 1/2 of 3aa, 3aq , and 3ua . 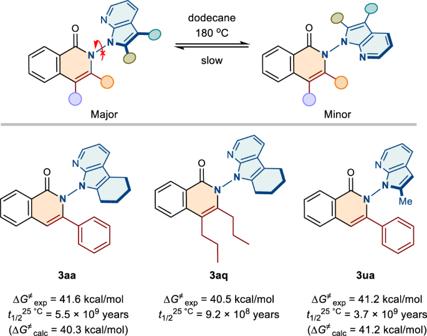Fig. 6: Study on product stability. The rotation barrier and thet1/2of3aa,3aq, and3ua. Full size image The gram-scale experiment using 1a (3.5 mmol, 1.02 g) with 2a under standard conditions delivered 3aa without obvious decrease in yield and enantioselectivity (88% yield, 96% ee). Furthermore, the annulation of 1a with diphenylphosphinoacetylene ( 2i ) on a gram-scale was caried out, leading to the formation of phosphoryl product 3ai with 60% yield and 99% ee (Fig. 7a ). The synthetic utility of this developed protocol to access N–N atropisomers was also further highlighted by post-functionalization. The compound 3ai was reduced to produce monophosphine product 4 with a remarkable 99% ee. In addition, the oxidative product 5 could be obtained by treatment of N-N axially chiral isoquinolinone 3aa with DDQ in 88% yield at 120 °C for 2 h. Further treatment of 5 with m -CPBA afforded N -oxide 6 . As the experimental result shown, the carbonyl group of N–N axially chiral isoquinolinone could also be easily transformed into a thiocarbonyl group in 75% yield without compromising enantioselectivity at the presence of Lawesson’s reagent (Fig. 7a ). Monophosphine product 4 could serve as a suitable chiral ligand for the asymmetric Pd-catalyzed allylic substitution reaction of indole and the Tsuji-Trost reaction, and the desired products were obtained with excellent yields and good to high enantioselectivities (73% ee for 8 , 93% ee for 9 ). In addition, N -oxide 6 was regarded as the chiral ligand to react with benzyl 2-diazo-2-phenylacetate and 1,2-dimethyl-1 H -indole in the presence of palladium catalyst to give desired 10 in 90% yield and 58% ee value (Fig. 7b ) [70] . Fig. 7: Gram-scale experiments and synthetic applications. a Gram-scale experiments using 1a as substrates and post-functionalization of N–N axially chiral product 3aa and 3ai . ee, enantiomeric excess; DDQ, 2,3-dichloro-5,6-dicyano-1,4-benzoquinone; m -CPBA, 3-chloroperoxybenzoic acid; BSA, N , O -bis(trimethylsilyl)-acetamide; DCM, dichloromethane; THF, tetrahydrofuran; rt, roomtemperature. b Applications of N–N axially chiral compound 4 and 6 as chiral ligands for further applications. Full size image To investigate the reaction mechanism, deuterium labeling experiments were conducted. H/D exchange experiments illustrated that the C-H cleavage was irreversible (Fig. 8a ). Then, the parallel and competitive kinetic isotope effect (KIE) values of 1.7 and 1.9 were calculated, indicating that C-H cleavage may be involved in the rate-determining step (Fig. 8b ). Furthermore, the study on the nonlinear effect between the enantiomeric excess (ee) of product 3aa and the ee of L6 revealed that a single chiral ligand coordinated with a cobalt atom to create an effective catalyst (Fig. 8c ). Based on the previous reports [65] , [66] , [67] , [68] , [69] , [70] , [71] , [72] , [73] and the above results, a plausible mechanism was proposed (Fig. 8d ). Cobalt salt (II) coordinates with L6 and AdCO 2 H, and undergoes oxidation with O 2 to produce active Co(III)-species A , which then undergoes ligand exchange with substrate 1a to form the octahedral Co(III)-intermediate B . The C–H activation of B affords the key intermediate C . It is worth mentioning that another pathway involving the first C-H activation step and the following oxidation step to form the intermediate C could not be completely ruled out. Next, alkyne 2a coordinates with C and the ligand exchange occurred to form D . The migration insertion of alkyne into the C-Co bond affords the seven-membered alkenyl intermediate E . Finally, the reductive elimination of E leads to the formation of the N–N axially chiral product 3aa and meanwhile releases the Co(I) intermediate F . Based on our previous report for the synthesis of C–N axially chiral compounds [70] , the reductive elimination through transition states TS-1 , which features the lowest-energy owing to the π - π stacking interactions between phenyl group of L6 with the 7-azaindole directing group of 1a , might serve as the enantio-determining step. Fig. 8: Mechanistic studies. a H/D Exchange experiments using 1a or [D 5 ]−1a as substrates. b Parallel and competitive kinetic isotope experiments to calculate KIE values. 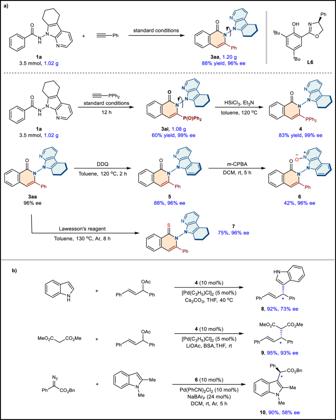Fig. 7: Gram-scale experiments and synthetic applications. aGram-scale experiments using1aas substrates and post-functionalization of N–N axially chiral product3aaand3ai. ee, enantiomeric excess; DDQ, 2,3-dichloro-5,6-dicyano-1,4-benzoquinone;m-CPBA, 3-chloroperoxybenzoic acid; BSA,N,O-bis(trimethylsilyl)-acetamide; DCM, dichloromethane; THF, tetrahydrofuran; rt, roomtemperature.bApplications of N–N axially chiral compound4and6as chiral ligands for further applications. 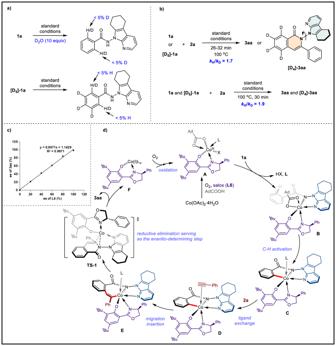Fig. 8: Mechanistic studies. aH/D Exchange experiments using1aor[D5]−1aas substrates.bParallel and competitive kinetic isotope experiments to calculate KIE values.cNolinear effect study between the enantiomeric excess (ee) of product3aaand the ee ofL6.dPlausible mechanism for the Co/Salox catalyzed annulation. c Nolinear effect study between the enantiomeric excess (ee) of product 3aa and the ee of L6 . d Plausible mechanism for the Co/Salox catalyzed annulation. Full size image In conclusion, we have developed an efficient and facile synthetic method for accessing N–N axially chiral isoquinolinones through cobalt-catalyzed atroposelective C–H activation/annulation. This protocol exhibits several unique characteristics, including a broad substrate scope, environmentally friendly O 2 as the oxidant, and excellent efficiencies and enantioselectivities. The obtained N–N axially chiral isoquinolinones features unique atropostability, which further expands the repertoire of N–N axially chiral derivatives. In addition, this method has proven to be a powerful strategy for constructing the N–N axial architectures under electrochemical conditions for asymmetric cobalt/Salox catalysis. Furthermore, other types of N–N axially chiral compounds, and related applications to asymmetric catalysis, functional materials are being evaluated in our laboratory and will be reported in due course. General procedure for the synthesis of compounds 3 An oven dried schleck tube charged with magnetic stirrer added benzamide/vinylamide 1 (0.2 mmol), Co(OAc) 2 ·4H 2 O (0.02 mmol, 10 mol%), L6 (0.04 mmol, 20 mol%), 1-adamantanecarboxylic acid (0.2 mmol, 1.0 equiv) with subsequent addition of 1,4-dioxane (2 mL) as solvent. To this reaction mixture, 2 (0.24 mmol, 1.2 eq) was added under O 2 . Then, the reaction system was stirred at 80 o C for 6 h. After the reaction was completed, the reaction mixture was quenched with saturated NaHCO 3 solution and extracted with CH 2 Cl 2 . The combined organic layer extracts were washed with brine, dried over Na 2 SO 4 , and concentrated under reduced pressure, and purified on silica gel chromatography (petroleum ether/ethyl acetate = 5:1) to afford the corresponding products. Full experimental details and characterization of the compounds are given in the Supplementary Information.